Whispering gallery microresonators for second harmonic light generation from a low number of small molecules Unmarked sensitive detection of molecules is needed in environmental pollution monitoring, disease diagnosis, security screening systems and in many other situations in which a substance must be identified. When molecules are attached or adsorbed onto an interface, detecting their presence is possible using second harmonic light generation, because at interfaces the inversion symmetry is broken. However, such light generation usually requires either dense matter or a large number of molecules combined with high-power laser sources. Here we show that using high-Q spherical microresonators and low average power, between 50 and 100 small non-fluorescent molecules deposited on the outer surface of the microresonator can generate a detectable change in the second harmonic light. This generation requires phase matching in the whispering gallery modes, which we achieved using a new procedure to periodically pattern, with nanometric precision, a molecular surface monolayer. Spherical or other circular microresonators exhibit high Q factors (quality factors) that result in very sharp resonances for the light that propagates in the so-called whispering gallery modes (WGM) [1] . In passive devices, small changes in the properties of the surface of the resonator would result in detectable displacements in the frequency of the resonant modes [2] , [3] , [4] , [5] . Recently, such displacements in the frequency of the resonant modes have been used to detect the presence of single molecules [6] , [7] or single viruses [8] . These results triggered the development of new theoretical work with the aim to fully elucidate the physical origin of such tiny displacements [9] . On the other hand, to enhance the sensitivity of such passive devices, it has been proposed that the alternative configurations based on a split-ring resonator be used to detect the presence of nanoparticles [10] , [11] . The combined use of a circular microresonator and a reference interferometer has also been considered to measure a wavelength shift produced by a nanoparticle as small as 1 fm (ref. 12 ). In all such cases, however, the passive nature of the underlying physics limits the applicability of the detection procedure to sense relatively large molecules or objects. In active devices, one may take advantage of the same high Q factors to obtain laser light generation [13] , [14] , [15] , [16] or to enhance nonlinear interactions [17] , [18] . In recent years, there has been some pioneering work with the goal to achieve efficient second or third harmonic generation [19] , [20] . This is, indeed, a challenging task because, in addition to having resonant modes at ω and 2 ω or 3 ω , one must phase match the two interacting waves. It has been theoretically shown that within circular microresonators, perfect phase matching may be achieved using different radial WGM for the fundamental and harmonic fields [21] , [22] , [23] , [24] , [25] . As shown in ref. 24 , phase matching amounts here to conservation of angular momentum. However, this happens only for specific radii and the overall overlap of the two interacting waves is limited. Quasi-phase matching is an alternative route that offers, in principle, more flexibility [21] , [24] but it was until now regarded as technically very difficult to implement. On the other hand, second harmonic generation (SHG) offers the possibility to interact with molecules that may be very small and those that do not emit light by fluorescence, molecules that are otherwise very difficult to detect. Yet the second-order interaction is extremely weak and the light emitted from such a type of molecule becomes detectable, in principle, only when a large number of molecules and large laser powers are used. Here we report the design and fabrication of a nonlinear spherical resonator to experimentally measure SHG from molecules deposited on its surface. Such nonlinear interaction was quasi-phase-matched by periodically patterning the surface molecular layer. Laser light pulses at the fundamental frequency were coupled into the whispering gallery modes of the high-Q spherical microresonators. By previously stretching the pulses to prevent walk-off, the interaction time could be increased up to several nanoseconds, provided the high Q factor of the microresonator. In other words, each molecule could be used many times to build up a light signal at the second harmonic (SH) frequency, and the number of molecules needed for the generation could be brought down to a level at which only 50–100 molecules were required to measure a detectable change in the generated light. Given that we used small non-fluorescent molecules, the proposed configuration opens the door to a very sensitive detection of label-free or unmarked very small molecules. Periodically patterned nonlinear spherical microresonator Crystal violet (CV) molecules were physically adsorbed on the surface of a micrometre-sized silica sphere, as described in the Methods section. This formed a low concentration monolayer of such molecules, which are non-fluorescent and very small. Each one of such molecules contains three aromatic rings to form a tetrahedron that occupies a volume of ∼ 0.02 nm 3 . To detect the presence of such a small quantity of material using SHG, it is advantageous when the molecules are placed on the surface of the microsphere in which the inversion symmetry is broken as required for a second-order nonlinear interaction in the dipole approximation. In addition, for WGM of the lowest radial order, the field is confined by the sphere surface around one equatorial plane. With such a monolayer, phase-matched SHG in the WGM would, in practice, be difficult to achieve except in some very specific conditions in which one can phase match the fundamental and second harmonic waves [24] . As explained in ref. 24, a more practical way to achieve phase matching in circular resonators would be to implement a periodic distribution of the nonlinear material on the surface. We proved that this is technically feasible using an electron beam gun. Indeed, by launching electrons accelerated under 10 kV, we were able to destroy the nonlinear activity of the organic molecules on the surface at will. To demonstrate the destruction of the nonlinear activity of the molecules, we first coated a flat surface with a 2.5×10 −4 M solution of CV and then exposed a strip of 1-mm width to the e-beam. 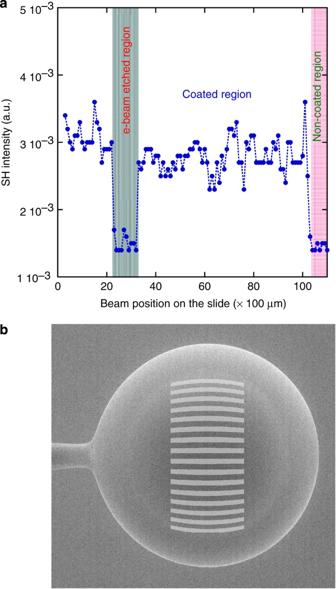Figure 1: Periodic molecular pattern on the sphere surface. (a) Second harmonic generation from a flat-surface substrate coated with a monolayer of nonlinear molecules. The SH intensity is shown as a function of the incident position of the beam on the substrate (blue dots). The dotted blue line is only a guide for the eye. The portion in which the nonlinear activity of the molecule was destroyed with the e-beam is shaded in grey, whereas the non-coated portion is shaded in red. (b) SEM image of the microsphere used in the experiment. The periodical pattern drawn on the sphere is superimposed on the SEM image of the sphere at the same scale. The diameter of the sphere was 359 μm. As shown in Figure 1a , we measured SHG from a laser beam focused down to a spot size of 100 μm in diameter, which we scanned over the 1-mm strip in which the nonlinearity of the molecule was destroyed by the e-beam. In this region, SH intensity drops down to the level obtained from the bare glass interface contribution. Further, we wrote a periodical pattern on roughly one quarter of the sphere around the equator, perpendicular to the stem that holds it, as shown in Figure 1b . The pattern consists of stripes, which must be exactly one coherence length wide. The design of this pattern must compensate both the material index dispersion and the modal effective index dispersion, which depends on the orbital number l . This number is related to the wavenumber in vacuum k and sphere radius a , as shown in the analytical expressions found in ref. 24 . 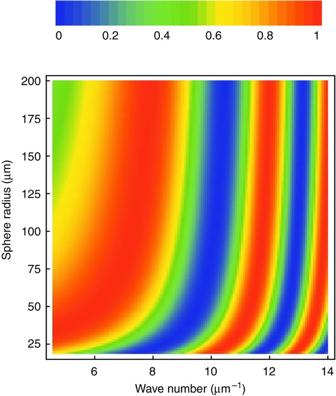Figure 2: Quasi-phased matching condition in the WGM of spheres. Equation (1) is given as a function of the radius of the sphere and wavenumber for the fundamental wave in vacuum. The arc length is fixed to 8.8 μm at the equator. In the fundamental WGM, the coupling between the amplitudes of the two interacting waves, κ , satisfies which is shown in Figure 2 as a function of k and a . In the above equation, L and l are the orbital numbers at the second harmonic and fundamental frequencies, respectively, whereas φ is the azimuthal angle. As seen in Figure 2 , when the radius of the sphere changes, the pattern indicating optimal conditions for SHG bends. This bending, which is more apparent when the sphere radius is small, is a consequence of the modal effective index dispersion. Along a latitude of polar angle θ on the surface of the sphere, the coherence length is As one moves away from the equator towards the poles, the coherence length becomes narrower, being maximum at the equator and zero at the poles. In other words, optimum quasi-phase matching is achievable when the periods resemble the curved surface of an orange slice. Such a periodic pattern of domains of width ℓ c , which is in the order of several micrometres, can be inscribed with 50-nm accuracy, using an electron beam. If the pattern of stripes on the sphere surface were to be projected on an equatorial plane perpendicular to the radius that passes through the centre of the central stripe, one would obtain a pattern as the one shown in white in Figure 1b . The coordinates of such projections were introduced into the SEM control unit to define the xy motion of the sphere (assuming that the xy plane is perpendicular to the e-beam). As long as the e-beam width remained constant and because of the sphere curvature, such xy motion produced on the sphere surface the desired pattern of stripes of equal length and width. To compensate for the e-beam divergence, we also moved the sphere in the z direction to ensure that the surface of the sphere always remained in focus with the e-beam. Following such procedure, the uncertainty when drawing the pattern was reduced to a minimum and the pattern inscribing became very reproducible. Note that the pattern drawn did not reach the poles (see Fig. 1b ), because, as shown in the Methods section, the interaction region for fundamental WGM is mostly confined around the equatorial plane. Drawing the pattern up to the poles would have no positive effect and would only increase the manipulation of the sphere resonator, which in the end would result in a reduction of the Q factor. Figure 1: Periodic molecular pattern on the sphere surface. ( a ) Second harmonic generation from a flat-surface substrate coated with a monolayer of nonlinear molecules. The SH intensity is shown as a function of the incident position of the beam on the substrate (blue dots). The dotted blue line is only a guide for the eye. The portion in which the nonlinear activity of the molecule was destroyed with the e-beam is shaded in grey, whereas the non-coated portion is shaded in red. ( b ) SEM image of the microsphere used in the experiment. The periodical pattern drawn on the sphere is superimposed on the SEM image of the sphere at the same scale. The diameter of the sphere was 359 μm. Full size image Figure 2: Quasi-phased matching condition in the WGM of spheres. Equation (1) is given as a function of the radius of the sphere and wavenumber for the fundamental wave in vacuum. The arc length is fixed to 8.8 μm at the equator. Full size image Surface SHG in the WGM To measure SHG, we used a tunable laser emitting a 1-kHz train of 150 fs pulses centred at 800 nm in wavelength. An average power of 200 μW of the train of pulses was coupled into an optical fibre. 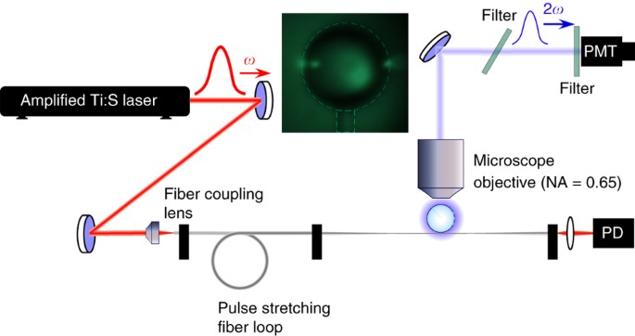Figure 3: Experimental setup. Schematic view of the experimental setup used for measuring the SH light generated by the nonlinear grating at the surface of the microsphere. The fibre loop is used only in the experiments in which the fundamental pulse is stretched to uniformly cover the entire perimeter of the sphere. The inset shows the polar and radial distribution of the WGM when the pulse is coupled into the microsphere (bright spot on the right). The picture was taken from a sphere doped with erbium atoms to facilitate the visibility of the WGM. The other two spots on the left correspond to images or parasitic reflections formed by the sphere of the residual light uncoupled from the taper to the sphere. PMT indicates photomultiplier tube. PD indicates photodetector. NA indicates numerical aperture. After travelling through the 1.5-m fibre used in the set-up, drawn schematically in Figure 3 , the pulses were lengthened to ∼ 1.1 ps. The fibre was tapered, and at the centre of such a tapered region, the diameter reached a minimum value of 1 μm. By bringing the sphere close to the centre of the tapered section, the light pulses were coupled into some of the fundamental WGM of the microsphere [26] , [27] . The radii of the majority of the spheres used in the experiments reported ranged from 177 to 183 μm. Directly from the spherical harmonics, corresponding to the fundamental beam given in the Methods section, we may determine the arc length of the fundamental field distribution inside the sphere to be close to 7.5 μm. This coincides very well with the experimentally measured one from the picture shown in the inset of Figure 3 . The generated second harmonic pulses at around 400 nm leaked out of the sphere because of Rayleigh scattering by defects on the sphere surface, and that light, after proper filtering, was detected using a reverse-biased photomultiplier tube (PMT). As seen in Figure 3 , to maximize the collection of the scattered light, we used a microscope objective with numerical aperture 0.65. In the Methods section, we describe the sensitivity of the setup in terms of the minimum number of photons required to measure upconversion. The first step to optimize the conversion efficiency in each experiment was to move the sphere along the taper, while SHG intensity was measured as a function of such a sphere position. By simultaneously measuring the transmission through the fibre and the SHG intensity, we observed that as the transmission diminished, indicating a more effective coupling of the fundamental field from the fibre to the sphere, the observed SH intensity increased. Maximum SHG thus corresponded to minimum transmission through the fibre. Figure 3: Experimental setup. Schematic view of the experimental setup used for measuring the SH light generated by the nonlinear grating at the surface of the microsphere. The fibre loop is used only in the experiments in which the fundamental pulse is stretched to uniformly cover the entire perimeter of the sphere. The inset shows the polar and radial distribution of the WGM when the pulse is coupled into the microsphere (bright spot on the right). The picture was taken from a sphere doped with erbium atoms to facilitate the visibility of the WGM. The other two spots on the left correspond to images or parasitic reflections formed by the sphere of the residual light uncoupled from the taper to the sphere. PMT indicates photomultiplier tube. PD indicates photodetector. NA indicates numerical aperture. Full size image The spheres we used in these experiments were coated, as described in the Methods section, from solutions of CV, the concentration of which ranged from 2.5×10 −4 to 1.55×10 −9 M. At concentrations above 2.5×10 −5 M, the Rayleigh-scattered SH light from the sphere surface was detectable using the set-up described above. 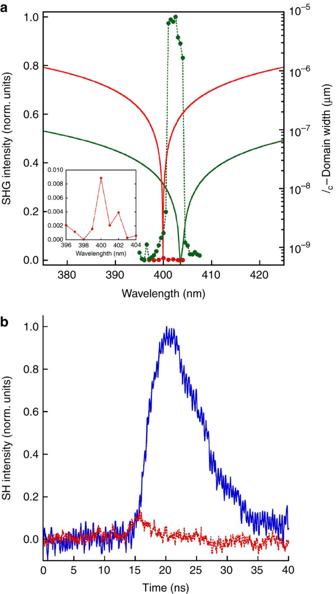Figure 4: Quasi-phase-matched SHG in the WGM. (a) Second harmonic generation as a function of half the wavelength of the fundamental wave when the coating solution was 2.5×10−4M (green dots) and when the coating solution was 5×10−9M (red dots). Experimental domain width minus the calculated coherence length at the equator as a function of half the wavelength of the fundamental wave in a logarithmic scale when the coating solution was 2.5×10−4M (green line) and when the coating solution was 5×10−9M (red line). The dashed lines are only a guide for the eye. The inset shows an enlarged view of the red dotted curve. The two experiments were performed using very similar spheres. The units of the vertical axis of the inset are the same as the left vertical axis of the main figure. (b) SH intensity as a function of time, using a sphere withQ=1.83×107(blue solid line) and a sphere withQ=3.72×106(red dotted line). Both spheres were coated with a 5.0×10−7M solution of CV and periodically patterned to achieve the phase-matching condition. All the parameters of the experimental setup, coupling taper, input intensity and so on were kept equal. The difference in Q factor must be attributed mostly to a difference in the eccentricity, whereas the difference in radius between the two spheres was only 16%. One in the vertical scale corresponds to an intensity current of 96 μA. As shown by the green dots of Figure 4a, by tuning the wavelength in a range between 790 and 820 nm, SHG strongly peaks at exactly 403 nm, very close to the quasi-phase-matching condition at 403.5 nm, predicted using equation 2 from the theory in ref. 24 . In this numerical application of the theory, we used no adjustable parameters and all the numbers used correspond to the actual parameters of the experiment or materials. The agreement is remarkable and the 0.5-nm displacement could be attributed to the slight shift in the resonances predicted by the analytical model [24] or a small error in measuring the diameter of the sphere. Note that, as indicated in ref. 24 , quasi-phase matching ensures that both waves propagate in resonant modes of the cavity. The light at the fundamental or second harmonic frequencies travels in more than one resonant mode of the cavity and consequently the conservation of energy is ensured within the bandwidth of the pulses used, which was ∼ 5 THz. Using a sphere with a Q =8.9×10 6 coated with a 2.5×10 −5 M solution of CV, we confirmed that the SHG dependence with the fundamental pumping intensity is quadratic. Indeed, we placed an NG5 filter that provides a 50% transmission at both 400 and 800 nm, first at the entrance of the coupling fibre and later in front of the PMT. In the first measurement, the SHG is reduced close to 25%, whereas in the last one the SHG is only reduced to 50%, confirming the quadratic behaviour of the SHG when using the spherical microresonator configuration described above. Figure 4: Quasi-phase-matched SHG in the WGM. ( a ) Second harmonic generation as a function of half the wavelength of the fundamental wave when the coating solution was 2.5×10 −4 M (green dots) and when the coating solution was 5×10 −9 M (red dots). Experimental domain width minus the calculated coherence length at the equator as a function of half the wavelength of the fundamental wave in a logarithmic scale when the coating solution was 2.5×10 −4 M (green line) and when the coating solution was 5×10 −9 M (red line). The dashed lines are only a guide for the eye. The inset shows an enlarged view of the red dotted curve. The two experiments were performed using very similar spheres. The units of the vertical axis of the inset are the same as the left vertical axis of the main figure. ( b ) SH intensity as a function of time, using a sphere with Q =1.83×10 7 (blue solid line) and a sphere with Q =3.72×10 6 (red dotted line). Both spheres were coated with a 5.0×10 −7 M solution of CV and periodically patterned to achieve the phase-matching condition. All the parameters of the experimental setup, coupling taper, input intensity and so on were kept equal. The difference in Q factor must be attributed mostly to a difference in the eccentricity, whereas the difference in radius between the two spheres was only 16%. One in the vertical scale corresponds to an intensity current of 96 μA. Full size image When the Q factor of the spheres used above ranged from 3.3×10 6 up to 6.9×10 7 , in the conditions described above, no SH signal could be detected for concentrations below 2.5×10 −5 M. Indeed, temporal walk-off between fundamental and SH pulses reduced the interacting length down to a very short distance, equivalent to having a Q factor of ∼ 10 4 . To take full advantage of the nominal Q factor, we stretched the pulses to a length that is equal or larger than the perimeter of the spheres used. We used 140 m of an optical fibre loop placed in between the entrance of the fibre and the tapered region, as schematically shown in Figure 3 . When the pulse reached the coupling region between the fibre and the sphere, it stretched up to ∼ 100 ps, the length of which is close to 21 times the perimeter of the largest sphere used in the experiments reported. As explained in more detail in the Methods section, the length of such a fibre loop was optimal because it had the added advantage that the unwanted visible white-light generation at the entrance tip of the fibre could be easily temporally filtered from the SH signal. After 140 m along the length of the fibre, when the visible portion of such white light centred at the SH frequency reached the coupling region, it was delayed by ∼ 22 ns with respect to the fundamental pulse. The combined effect of pulse stretching and temporal filtering in the fibre improved the signal detection efficiency by four to five orders of magnitude. Using spheres with a nominal Q factor of 2.4×10 7 , we were thus able to measure the quasi-phase-matched SHG peak, shown as red dots in Figure 4a , from a sphere coated with a 5×10 −9 M solution of CV. When performing high-sensitivity measurements using CV solutions at concentrations equal or below 5×10 −9 , one had to find a trade-off between a high level of pumping intensity to increase the efficiency of the SHG from CV, and a lower pumping level to prevent the onset of other unwanted nonlinear processes, such as white-light generation at the tapered portion of the fibre or light-induced damaging of the fibre entrance tip. This leaves a window for the pump-power level, which is narrowed down as the molecular surface concentration is decreased. For the lowest molecular concentration that we measured, the optimal pump energy corresponded to ∼ 0.025 nJ per pulse. The role that the Q factor had in the efficiency of the SHG process was evaluated by comparing the SH intensity when two different spheres with different Q factors were used as microresonators. It is important to note that the experimental conditions for the two experiments were maintained exactly the same. As may be seen in Figure 4b , a comparison of the integrated SH intensity over time indicates that a 4.9 times increase in the Q factor resulted in an increase in the energy conversion by a factor of 25, slightly larger than Q 2 . This clearly demonstrated the positive effect brought to the nonlinear interaction by the light localization within the microresonator. The build-up of intensity at the SH frequency is significantly more effective when the Q is larger. In other words, as one would have expected, there is an increase in the total dwell time for the SH light pulse; however, there is also an increase, larger than seven times, in the maximum SH intensity measured, as shown in Figure 4b . Using a new pair of microspheres, we repeated the experiment, but reducing the CV coating concentration molarity by a factor of 100. We observed that a 3.6 times increase in the Q factor led to a 19.1 times increase in the SH energy conversion, again less than Q 3 but larger than Q 2 . This confirmed the relevant role of the Q factor. Using the coupled mode approach developed in ref. 24 , we analytically determined the role of the sphere Q factor on the SHG. To this end, following ref. 24 , we denote the field amplitudes of the fundamental and second harmonic WGM by α 1 and α 2 , respectively. With the appropriate choice of units, ( ω / Q 1 )| α 1 | 2 is the power lost by the fundamental mode by linear processes, ω is the fundamental frequency and Q 1 is the associated quality factor. Besides the natural far-field radiation of WGM from perfect spheres, decay channels include Rayleigh scattering from surface imperfections, parasitic absorption or out-coupling to neighbouring waveguides. Similarly, (2 ω / Q 2 )| α 2 | 2 is the power lost by the second harmonic mode and a fraction of it is collected as a usable signal. Given the optical power P taper in the taper fibre and an out-coupling Q factor Q o , energy is injected in the fundamental mode at a rate of P taper / Q o at resonance. Equilibrium is thus reached when ( ω / Q 1 )| α 1 | 2 = P taper / Q o . On the other hand, standard couple-mode theory dictates that ( ω / Q 2 + i Δ) α 2 = iκ | α 1 | 2 , where Δ is the frequency mismatch between the fundamental and second harmonic. Eventually, therefore, the out-coupled SHG intensity is proportional to Hence, when energy is conserved Δ=0, and assuming that Q 1 = Q 2 = Q we expect the SHG signal to scale as Q 3 in optimal conditions. The fact that we experimentally measure a proportionality below Q 3 may be attributed to small variations in the coupling conditions when different spheres are used, which eventually results in a change in the Q o factor. Number of molecules for SH light generation To study the sensitivity of SH signal to CV concentration, we performed a set of experiments to determine the SHG dependence on the concentration of molecules, using four different CV concentration solutions ranging from 5×10 −9 up to 5×10 −6 M. To avoid dispersion in the diameter or Q factors, we performed the experiment using only one sphere that we coated starting with the smallest concentration and writing the grating and then performing the SH measurement. Subsequently, we repeated this procedure three times, each time with a concentration that was ten times larger than the previous one. 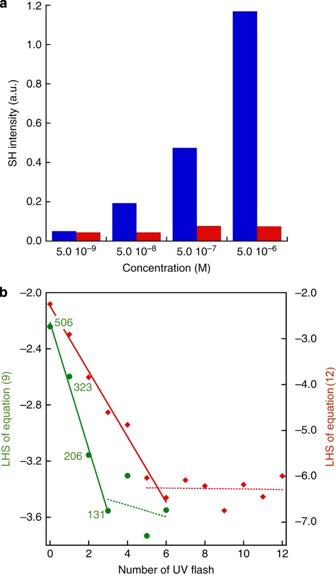Figure 5: Sensitivity to molecular concentration or number. (a) Second harmonic signal in arbitrary units (a.u.) for four different surface concentrations of nonlinear molecules when a grating was written (blue bars) and when no grating was written (red bars). In the horizontal axis, we indicate the concentration of the original solution used to prepare the monolayers. (b) Left hand side of equation (9) in which the variables correspond to the experimentally measured intensities (vertical axis). Sequence of 1-s ultraviolet (UV) flashes (horizontal axis). The background noise is subtracted from the measured intensity and then this difference is divided by the reference input intensity to ensure a unit less logarithm argument and proportionality to the molecular surface density. Two different spheres were coated with a 1.55×10−9M solution of CV (green dots) and with a 1×10−7M solution of CV (red dots). Given different conditions in the two experimental measurements, which use two different spheres, one should not expect the two decreasing slopes to be identical. The numbers shown by the green dots obtained using equation (7) should not be taken literally and are only indicative of the molecules that participate in the SHG before shining each ultraviolet flash. The solid lines indicate a linear adjustment to the portion of data that shows a decrease, whereas the dotted lines indicate a linear adjustment to the almost horizontal portion of the data. As shown in Figure 5a , the SH signal increases with increasing concentration, with a growth rate that deviates from the quadratic growth rate that one would expect. It is not clear what the origin of the SHG efficiency saturation is as the CV concentration increases. One possibility could be a small degradation in the Q factor after the coating procedure is repeated each time. For instance, we observed a 20% decrease of the Q factor when the sphere was coated with a 5×10 −7 M solution of CV. Molecular absorption alone, however, could not account for the slow growth rate observed in Figure 5a . Possibly, another less controllable source that lowers the Q factor each time a new grating is inscribed may also exist. A discrepancy could also arise from a degradation of the quasi-phase-matching condition caused by the residual molecules from the previous coating, leading to a shallower grating. However, provided that no other change is introduced except for a change in the number of molecules, the proportionality relation , N being the number of molecules, must hold, as in the ultraviolet flash lamp experiments reported below in which nothing in the experimental setup was modified during the course of the experiment. We also measured SH from a similar sequence in which we did not perform the grating in any of the steps. As seen in Figure 5a , the SH signal measured in those cases was down to noise level at all concentrations. This shows that in detection devices based on the results reported, it would be very simple to discriminate the molecule to be detected from any other molecule that could attach to the surface even if such an unwanted molecule is a better SH generator. Following a patterned functionalization, only the molecule to be detected would end up in the periodic pattern required for quasi-phase matching. Figure 5: Sensitivity to molecular concentration or number. ( a ) Second harmonic signal in arbitrary units (a.u.) for four different surface concentrations of nonlinear molecules when a grating was written (blue bars) and when no grating was written (red bars). In the horizontal axis, we indicate the concentration of the original solution used to prepare the monolayers. ( b ) Left hand side of equation (9) in which the variables correspond to the experimentally measured intensities (vertical axis). Sequence of 1-s ultraviolet (UV) flashes (horizontal axis). The background noise is subtracted from the measured intensity and then this difference is divided by the reference input intensity to ensure a unit less logarithm argument and proportionality to the molecular surface density. Two different spheres were coated with a 1.55×10 −9 M solution of CV (green dots) and with a 1×10 −7 M solution of CV (red dots). Given different conditions in the two experimental measurements, which use two different spheres, one should not expect the two decreasing slopes to be identical. The numbers shown by the green dots obtained using equation (7) should not be taken literally and are only indicative of the molecules that participate in the SHG before shining each ultraviolet flash. The solid lines indicate a linear adjustment to the portion of data that shows a decrease, whereas the dotted lines indicate a linear adjustment to the almost horizontal portion of the data. Full size image To discover the absolute sensitivity of the surface SHG in the microspheres, we report here an experiment that we performed to estimate the minimum number of molecules that are required to measure a change in the SH signal. We measured the SH signal decrease after subsequent 1-s ultraviolet flashes from a disinfection ultraviolet lamp, with an intensity peak at 253.7 nm, were shone on the sphere to photodegrade the CV. We considered two different spheres coated with two different concentrations. As seen in Figure 5b , the square root of the normalized corrected SH intensity (see left hand side of equation (9) from the Methods section) displayed a similar behaviour in both cases. One sees a relatively fast exponential decay, followed by an almost non-decaying signal that is down to the noise level. Using the slope determined from Figure 5b and equation (7) in the Methods section, we can accurately estimate the number of molecules that are required to see a measurable change in SHG. The smallest concentration of the two considered in Figure 5b was (1.55±0.04)×10 −9 M, which leads to a CV density on the sphere surface of (7.90±0.14)×10 7 molecules per cm 2 . The Q =8.67×10 7 for that sphere was the largest value that was used in all the experiments reported. As determined in the Methods section, the total number of molecules that contribute to SHG is ∼ 506±9. As shown in Figure 5b , after the first ultraviolet flash, the total number of molecules available for SHG reduces to 323, after the second to 206 and after the third one to 131. In the last step, the nonlinear activity of 75 molecules was destroyed by the ultraviolet flash. After that third flash the signal is down to the noise level. Provided that the noise measured from the non-decaying portion of the data would correspond to a molecule number dispersion close to 50, we may conclude that ∼ 50–100 molecules are needed to detect a measurable change in SHG. Similarly, we can determine the sensitivity when the sphere is coated with a 10 −7 M concentration of molecules. For such a larger concentration, as discussed in reference to the results reported in Figure 5a , the sensitivity is lower. Sensing of label-free or unmarked molecules could be one of the major fields of application for the type of quasi-phase-matched SHG in the WGM in spherical microresonators we propose. With such a resonator configuration, to obtain a measurable SH signal one needs a molecular surface density ∼ 10,000 times lower than when SHG is measured directly from a flat surface under similar pumping conditions. The role of the cavity in the resonator case was clearly confirmed when the enhancement ratio provided by the resonator was measured to scale between Q 2 and Q 3 . When we consider the total number of molecules, to obtain a measurable signal, one needs at least 4×10 6 molecules in the flat-surface configuration, as opposed to 50–100 for the resonator case, in which the molecules only detect the evanescent tail of the field stored in the microresonator. Note that, for the flat-surface configuration, a high pumping intensity directly hitting the molecules causes a rapid degradation, which does not occur in the resonator case. Earlier configurations based on microresonators to detect single objects could not be used to detect small molecules, even if a large number were to be used. Such configurations are based on producing a local change on the surface of the microresonator, and this is only possible if one uses large molecules or tens of nanometre-sized particles. Consequently, the potential for applications in sensing for the physical phenomenon reported here is very different and complementary to those alternative approaches. The particular setup of the configuration we proposed, in which molecules assemble at an interface at which the interaction is enhanced by the large Q factors available, opens up the possibility to obtain an efficient SHG from any type of molecules, even if they are centrosymmetric or if the dipole moment in the ground state is zero, as for the molecule used. In other words, any kind of label-free, large or small molecule is, in principle, detectable. We have also demonstrated experimentally that the nonlinear activity of organic molecules deposited on a spherical surface could be erased using an electron beam, which allowed us to write the exact periodic pattern we needed for quasi-phase matching. The periodic quasi-phase-matched SHG implemented here has the added value that contributions from the bulk or the non-patterned interface are essentially negligible, as they are, in general, not phase matched unless some very particular requirements for the set of parameters that define the microresonator are met. We have also shown that SHG in the microresonator configuration considered provides a means for temporal walk-off compensation when the interacting pulses are longer than the resonator perimeter. The quasi-phase-matched SHG experimental demonstration reported is the first step to many other parametric process and opens up the possibility to study experimentally phase-matched quadratic NL optics in any circular high-Q cavity configuration that remained, until recently, very much unexplored. Molecular surface layer preparation and density CV molecules were dissolved in a 1-propanol solution in which the entire sphere and the stem that holds it were immersed. These were removed from the solution at a constant speed of 1 mm s −1 using a motorized translation stage. This produces a very homogenous monolayer coating with a surface density that is linearly proportional to the concentration of CV in the solution. To eliminate solvent residues, the sphere was dried in a furnace at 50 °C for 10 min. Given the proportionality between the CV surface density and concentration in solution, we may accurately determine the number of molecules participating in the interaction, as described below. Using a high-sensitivity ultraviolet/visible spectrophotometer and a 1-cm path-ength cell, we measured the absorption spectrum of the lowest CV concentration in solution for a detectable SH signal. We determined it to be (1.55±0.04)×10 −9 M, provided that the CV cross-section in 1-propanol at 596 nm was (11.5±0.3)×10 −16 cm 2 . We accurately measured such a cross-section using five independently prepared 10 −7 M solutions of CV in 1-propanol. Thus, the CV density on the surface sphere for this concentration was (7.90±0.14)×10 7 molecules per cm 2 . Sensitivity in measuring the scattered SH light Each SHG measurement shown in the figures corresponds to the result of averaging the SH signal obtained from 10,000 laser pulses. As an example, the area under the blue solid curve from Figure 4b is proportional to the energy or number of photons at the SH frequency. Taking into account the PMT-cathode sensitivity and gain, the conversion from the intensity current-time integral to energy indicates that for each pulse ∼ 50 photons were detected. In the same Figure 4b , the red dotted line would correspond to approximately two photons per pulse. This would correspond to two spikes above the base line, which, most likely, would not be visible because of the dark current noise. However, the SH signal could be made apparent because the curve shown corresponds to, as mentioned above, the averaging of 10,000 pulses, in other words, to the detection of ∼ 20,000 photons. This is roughly the limit of the measuring system used in terms of the photons needed to obtain a signal above the noise level. However, this does not set a limit on the number of molecules needed for a measurable SHG. By optimizing the setup, essentially by increasing the Q factor of the sphere, we were able to lower the concentration of the CV coating solution by more than two orders of magnitude as reported. In the results shown in Figure 5b , the detection of 506 molecules corresponds approximately to the detection of two to three photons per pulse, 323 molecules to two photons per pulse and 206 to one to two photons per pulse. Pulse stretching and continuous wave pumping To achieve an optimal pulse walk-off, we tested four different fibre lengths. The results obtained are summarized in Table 1 . In all four cases, the SH signal was monitored while scanning the wavelength of the input laser within the 100-nm range of tunability of the amplified laser system used. The CV coating concentration used was 1×10 −8 M, whereas the sphere Q factor was 3.82×10 7 . For the 1.5-m fibre, the pulse intensity remained the largest one, 12.2% relative to the intensity of the original non-stretched pulse. However, no phase-matching peak could be observed because the SH signal from the molecules overlapped with the white light generated at the pulse entrance tip of the fibre, combined with the fact that a pulse length shorter than the perimeter of the microresonator cavity prevented pulse walk-off compensation. When the pulse was stretched up to 10.7 ps, corresponding to close to twice the pulse roundtrip time within the resonator, we still did not observe any phase-matching peak. In that case, the delay between the fundamental pulse and white light was only 1.58 ns (ref. 28 ). Proper temporal filtering from the white light was not possible, provided the large Q resulted in a signal lifetime close to 7 ns. Using a 140-m fibre, we introduced a delay time equivalent to 22.2 ns between the fundamental and white light pulses. Such delay was sufficient to temporally separate the SH signal from such white light. A proper separation requires a delay of about three times the decay time of the SH signal, which in the majority of measurements we performed ranged between 6 and 8 ns. In addition, the pumping pulse was stretched close to 20 times the equator length and walk-off could be perfectly compensated. Further improving of the sensitivity could be reached by slightly increasing the intensity of the laser input pulse, as indicated above in the main text. Additional stretching of the pulse to reach a larger delay, which would be needed if very large Q factor spheres were to be used, proved to be unsuccessful. The failure in measuring a phase-matching SH peak could be attributed to a weak intensity at the tapered region equivalent to 0.046% of the incident pulse intensity. In summary, the 140-m fibre length proved to be optimal, which also allowed us to test spheres with Q factors that are slightly larger. Table 1 SHG performance for four different lengths of the pulse-stretching fibre loop. Full size table We also leveraged the performance of the pulse configuration against the continuous wave (CW) excitation using 250-mW CW laser power tuned at ∼ 800 nm. When coupling this power into the sphere, we did not measure any SH response. Comparing the peak intensities that we could reach inside the sphere in the CW case (10 7 W cm −2 ) relative to the one that we could reach in the pulsed case (10 10 W cm −2 ) may provide an explanation as to why we were not able to see any signal in the CW case. Most probably, when the entire procedure of sphere fabrication, monolayer deposition and periodical patterning can be carried out on microresonators with Q factors of 10 9 , surface SHG in CW might be possible too. Using pulses has some disadvantages but also some advantages, one of them is that several ' l ' modes of the sphere are excited, and further phase matching simultaneous to energy conservation does not become an improbable task. In other words, strictly speaking, within the pulse, we may use three different resonance modes to have sum frequency with a very small detuning from perfect SHG. It is also likely that such an energy conservation may be eased by the Kerr nonlinearity, as it was proposed in ref. 17 . Number of molecules To estimate the total number of molecules participating in the interaction, we must consider the total number of coated stripes on the sphere surface and the interaction area within each stripe. Such an area is equal to the product of the equatorial length of the stripe times the interaction length in the polar direction. To determine such a length in the polar direction, we use the expression deduced from ref. 24 . For fundamental WGM, which are concentrated on the equator, we have M = L , m = l and Provided that χ is proportional to the surface density of molecules ρ ( θ , φ ), equation (4) becomes Similar expressions could be derived for all the coupling constants found in ref. 24 . The integrand above leads to an effective density that is halved when On the other hand, L ∼ 2n 2 ka = 4 π n 2 a/λ and l ∼ n 1 ka = 2 π n 1 a/λ , where λ is the fundamental wavelength. The effective arc length in the θ direction is, therefore: Assuming a =177 μm, λ =0.8 μm, n 1 =1.45 and n 2 =1.47, this yields s =4.6 μm. As the length of the stripe at the equator in the azimuthal direction is equal to 8.7 μm and the total number of stripes on the sphere used is 16, in the SH measurements shown in Figure 5b , the total number of molecules participating in the interaction at the starting point, before any ultraviolet flash was shone, was ∼ 506±9. After shining a ultraviolet flash lasting for a time d t , the number of molecules on the surface decreases as where N is the number of molecules, I uv is the ultraviolet intensity at the sphere surface and α is a constant of proportionality to maintain the units correct. After integration with respect to time, the number of molecules is given by where N o is the initial number of molecules and α ′= αI uv . By using equation (7) and the direct proportionality of the intensity of the SHG light to the square of the number of molecules, the measured SH intensity at a given time may be written as where I bg is the background signal noise at the SH frequency not coming from the molecules, β is a constant and I ω is the fundamental pump intensity. If we normalize such a measured SH intensity to the intensity of the incident fundamental field, then the following linear relation must hold The experimental values for the left hand side of equation (9) are plotted as a function of the ultraviolet flash number in Figure 5b . The value of α ′ is extracted from the slope and used in equation (7) to estimate the number of molecules remaining after each ultraviolet flash is shone. How to cite this article: Dominguez-Juarez, J.L. et al . Whispering gallery microresonators for second harmonic light generation from a low number of small molecules. Nat. Commun. 2:254 doi: 10.1038/ncomms1253 (2011).